SUMO2/3 modification of cyclin E contributes to the control of replication origin firing The small ubiquitin-like modifier (SUMO) pathway is essential for the maintenance of genome stability. We investigated its possible involvement in the control of DNA replication during S phase by using the Xenopus cell-free system. Here we show that the SUMO pathway is critical to limit the number and, thus, the density of replication origins that are activated in early S phase. We identified cyclin E, which regulates cyclin-dependent kinase 2 (Cdk2) to trigger origin firing, as an S-phase substrate of this pathway. We show that cyclin E is dynamically and highly conjugated to SUMO2/3 on chromatin, independently of Cdk2 activity and origin activation. Moreover, cyclin E is the predominant SUMO2/3 target on chromatin in early S phase, as cyclin E depletion abolishes, while its readdition restores, the SUMO2/3 signal. Together, our data indicate that cyclin E SUMOylation is important for controlling origin firing once the cyclin E–Cdk2 complex is recruited onto replication origins. Post-translational modifiers of the small ubiquitin-like modifier (SUMO) family have emerged as key regulators of protein function and fate. SUMOylation , which is the covalent and reversible conjugation of SUMO to target proteins, is essential for growth, division and maintenance of genome stability from yeast to mammals. Among the many functions of SUMO modification are regulation of transcription, DNA repair, nuclear transport and formation of sub-nuclear structures [1] , [2] , [3] , [4] , [5] , [6] , [7] , [8] . Three SUMO isoforms (~100 amino-acid proteins) are expressed in vertebrates: SUMO1, SUMO2 and SUMO3. SUMO2 and 3 are highly related and both contain a SUMO consensus modification motif that allows the formation of polySUMO chains, and is absent in SUMO1. SUMOylation occurs via a biochemical pathway that is analogous to the ubiquitylation cascade, but with a distinct set of enzymes: the E1 SUMO-activating enzyme (SAE1/SAE2), the E2-conjugating enzyme (Ubc9) and, at least in some cases, additional E3 ligases. The first evidence of a connection between SUMO and DNA replication and repair came from the discovery that proliferating cell nuclear antigen (PCNA), the DNA polymerase processivity factor, can be conjugated with SUMO at the replication fork [9] . PCNA SUMOylation has been reported in yeast, Xenopus and recently in mammalian cells, and it appears to occur during S phase under physiological conditions [9] , [10] , [11] . However, even in yeast, SUMOylation of PCNA is hard to detect because only a small proportion of PCNA is modified. In addition, lack of PCNA SUMOylation does not lead to a striking phenotype during normal growth in yeast, suggesting that it is not essential for replication in undamaged cells. However, in response to DNA damage, PCNA is strongly SUMOylated on chromatin to facilitate the recruitment of Srs2 at stalled replication forks and thereby block inappropriate recombination [12] . Recent studies revealed that in addition to PCNA, many proteins involved in DNA replication and repair are SUMOylated in response to heat stress and DNA damage, highlighting the fact that defects in SUMOylation might impair replication of damaged DNA [13] , [14] , [15] . In the present study, we investigated the impact of SUMOylation on the control of DNA replication in unchallenged conditions in a cell-free replication system. Our findings show that SUMOylation is critical for the prevention of excessive origin firing and extend the number of known SUMO substrates with the identification of cyclin E, a key actor in origin activation, as the most likely candidate for mediating this regulation. SUMOylation controls replication origin density We used the Xenopus laevis egg extract system to investigate the role of the SUMO pathway in the control of DNA replication. When demembranated sperm nuclei are added to interphase egg extracts, sperm chromatin is first assembled into functional nuclei in about 30 min and then undergoes a single complete round of DNA replication [16] , [17] . We inhibited SUMOylation by adding Ubc9dn, a dominant-negative form of Ubc9 (ref. 18 ), to these extracts. Ubc9dn did not affect nuclei formation, in agreement with previously reported results [19] , but reproducibly increased the rate of DNA replication early in S phase in comparison with control extracts (without Ubc9dn) ( Fig. 1a ). A similar effect was also observed upon addition of a recombinant SUMO-specific protease that can remove SUMO moieties from SUMO-modified substrates (data not shown). To understand this effect, we then examined the pattern of replication origin firing at the beginning of S phase by combing replicating DNA from sperm nuclei. To this aim, we labelled early firing replication origins by adding 5-bromo-2′-deoxyuridine 5′-triphosphate (BrdU) to the extracts in the presence of sperm chromatin. Analysis of samples collected at the 30-min time-point after addition of sperm chromatin showed a significant increase in the frequency of initiation events in the presence of Ubc9dn, compared with control extracts (mean of 67.72/Mb versus 45.74) ( Fig. 1c ). Addition of Ubc9dn resulted in shorter inter-origin distances (IOD; mean IOD: 14.84 versus 22.06 kb) and shorter intervals between BrdU tracks (mean DNA gap size: 8.28 versus 15.02 kb), whereas it moderately affected the length of BrdU tracks (mean length: 6.96 versus 7.77 kb) ( Fig. 1e ). These results demonstrate that the higher replication rate observed at 30 min was due in large part to a higher number of initiation events. Similar results were obtained at 40 min ( Supplementary Fig. S1 ). Quantification of the data showed that inhibition of SUMO conjugation led to the activation of roughly 30–50% additional replication origins, compared with non-inhibited controls, demonstrating that the SUMO pathway has a critical negative role in controlling origin density in this system. 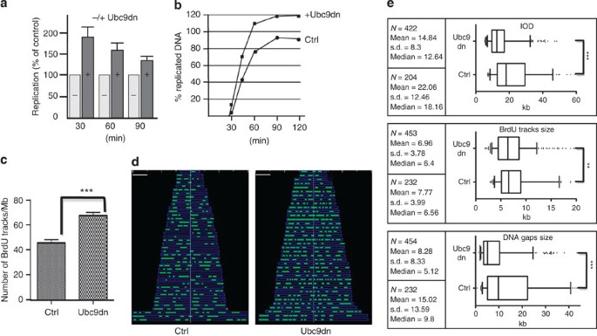Figure 1: Effect of Ubc9dn on origin firing in early S phase. (a) Sperm nuclei (2,000 nuclei per μl) were replicated inXenopusegg extracts supplemented (+) or not (−) (Ctrl, control) with 350 ng μl−1Ubc9dn. At each time-point after addition of sperm nuclei, DNA replication in samples with Ubc9dn was defined relative to that in Ctrl samples (set at 100%). DNA replication was measured by standard [33P]-labelled dCTP incorporation; mean±s.d. % Of DNA replicated in nine independent experiments based on four different egg extracts that replicated 90–100% of the input DNA. (b) Time-course of DNA replication in S-phaseXenopusegg extracts with or without Ubc9dn. The graph represents the percentage of input DNA that is replicated at each indicated time-point. (c) Quantification of the number of initiation events (number of BrdU tracks per Mb) on combed DNA fibres from the 30-min time-point with or without Ubc9dn of the replication reaction shown inb. (d) Distribution of initiation events on combed DNA fibres at the 30-min time-point. BrdU tracks are represented in green (bar, 50 kb). This representation was generated by using the IDeFIx software. (e) IOD, length of BrdU tracks and of DNA gaps between tracks measured for each condition (with or without Ubc9dn) at the 30-min time-point. Boxes and whiskers indicate the 5–95 percentiles. The vertical line within the boxes represents the median (in kb). Data not included between the whiskers are plotted as outliers (dots). Statistical significance was determined using the unpairedt-test (**P<0.001 and ***P<0.0001). Figure 1: Effect of Ubc9dn on origin firing in early S phase. ( a ) Sperm nuclei (2,000 nuclei per μl) were replicated in Xenopus egg extracts supplemented (+) or not (−) (Ctrl, control) with 350 ng μl −1 Ubc9dn. At each time-point after addition of sperm nuclei, DNA replication in samples with Ubc9dn was defined relative to that in Ctrl samples (set at 100%). DNA replication was measured by standard [ 33 P]-labelled dCTP incorporation; mean±s.d. % Of DNA replicated in nine independent experiments based on four different egg extracts that replicated 90–100% of the input DNA. ( b ) Time-course of DNA replication in S-phase Xenopus egg extracts with or without Ubc9dn. The graph represents the percentage of input DNA that is replicated at each indicated time-point. ( c ) Quantification of the number of initiation events (number of BrdU tracks per Mb) on combed DNA fibres from the 30-min time-point with or without Ubc9dn of the replication reaction shown in b . ( d ) Distribution of initiation events on combed DNA fibres at the 30-min time-point. BrdU tracks are represented in green (bar, 50 kb). This representation was generated by using the IDeFIx software. ( e ) IOD, length of BrdU tracks and of DNA gaps between tracks measured for each condition (with or without Ubc9dn) at the 30-min time-point. Boxes and whiskers indicate the 5–95 percentiles. The vertical line within the boxes represents the median (in kb). Data not included between the whiskers are plotted as outliers (dots). Statistical significance was determined using the unpaired t -test (** P <0.001 and *** P< 0.0001). Full size image S-phase SUMO2/3 conjugates depend on cyclin E presence We next analysed by western blotting the SUMOylation profile of S-phase targets in Xenopus egg extracts at 0 and 60-min after addition of sperm chromatin and Ubc9dn, or not (control). At the 60-min time-point, high-molecular-weight SUMO2/3 conjugates were easily detected in control egg extracts, but not when the replication assay was carried out in the presence of Ubc9dn ( Fig. 2a ). 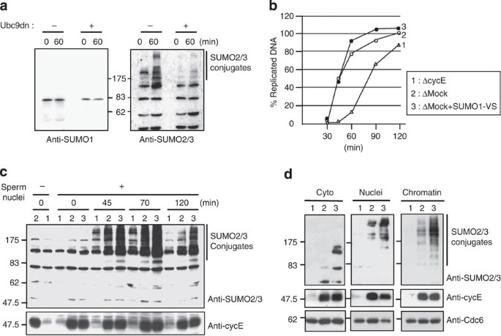Figure 2: Accumulation of SUMO2/3-conjugated proteins on chromatin during S phase depends on cyclin E. (a) S-phaseXenopusegg extracts were supplemented or not with Ubc9dn, as inFig. 1. The presence of SUMO-conjugated proteins was analysed by western blotting with anti-SUMO1 and anti-SUM02/3 antibodies, using replicating samples at the 60-min time-point. (b) Time-course of DNA replication in S-phaseXenopusegg extracts immunodepleted with anti-cyclin E (1) or control antibodies (2) or with Ctrl antibodies and supplemented with 5 μM SUMO1-VS (3), in the presence of α-[33P]-dCTP. The graph represents the percentage of input DNA replicated at each indicated time-point. (c)Xenopusegg extracts described inFig. 2b(2 μl) were immunoprobed with anti-SUMO2/3 and anti-cyclin E antibodies before addition of sperm nuclei and throughout the replication assays in cyclin E-depleted extract (1), control-depleted extract without (2) or with SUMO1-VS (3). (d) Aliquots of cytosol (Cyto), nuclei and chromatin fractions, corresponding to 2, 5 and 20 μl of extracts, respectively, were taken at the 45-min time-point after the addition of sperm nuclei from the replication reactions 1, 2 and 3, described inFig. 2band were immunoprobed with antibodies against SUMO2/3, cyclin E and Cdc6 (loading Ctrl). Figure 2: Accumulation of SUMO2/3-conjugated proteins on chromatin during S phase depends on cyclin E. ( a ) S-phase Xenopus egg extracts were supplemented or not with Ubc9dn, as in Fig. 1 . The presence of SUMO-conjugated proteins was analysed by western blotting with anti-SUMO1 and anti-SUM02/3 antibodies, using replicating samples at the 60-min time-point. ( b ) Time-course of DNA replication in S-phase Xenopus egg extracts immunodepleted with anti-cyclin E (1) or control antibodies (2) or with Ctrl antibodies and supplemented with 5 μM SUMO1-VS (3), in the presence of α-[ 33 P]-dCTP. The graph represents the percentage of input DNA replicated at each indicated time-point. ( c ) Xenopus egg extracts described in Fig. 2b (2 μl) were immunoprobed with anti-SUMO2/3 and anti-cyclin E antibodies before addition of sperm nuclei and throughout the replication assays in cyclin E-depleted extract (1), control-depleted extract without (2) or with SUMO1-VS (3). ( d ) Aliquots of cytosol (Cyto), nuclei and chromatin fractions, corresponding to 2, 5 and 20 μl of extracts, respectively, were taken at the 45-min time-point after the addition of sperm nuclei from the replication reactions 1, 2 and 3, described in Fig. 2b and were immunoprobed with antibodies against SUMO2/3, cyclin E and Cdc6 (loading Ctrl). Full size image The covalent attachment of SUMO moieties to proteins is a very dynamic process because of the action of SUMO-specific proteases (SENP) [20] , [21] , [22] . In addition, in the Xenopus cell-free system, cyclin-dependent kinase 2 (Cdk2) is associated exclusively with cyclin E, and cyclin E–Cdk2 complexes provide most of the Cdk activity necessary to drive replication initiation throughout S phase [23] , [24] , [25] . Thus, we examined SUMO2/3 conjugation at different time-points during replication in Xenopus egg extracts that lacked Cdk2 (due to cyclin E immunodepletion) or SENP activities (by supplementing the extracts with SUMO1-Vinyl Sulfone (SUMO1-VS), a specific and irreversible SENP1/2 inhibitor [22] ). Time-course analysis of DNA replication in such extracts showed that immunodepletion of cyclin E (>90%) caused a significant delay in DNA replication, although 80% of DNA synthesis was completed in 2 h, indicating that some origins were activated. Conversely, addition of SUMO1-VS did not affect the efficiency of DNA replication ( Fig. 2b ). Western blot analysis of the same samples showed that, whereas the presence of high-molecular-weight SUMO2/3 conjugates was exclusively dependent on the addition of sperm chromatin (data not shown), their amount at each time-point was strongly reduced in cyclin E-depleted extracts. In contrast, the amount of conjugates was significantly enhanced in the presence of the SENP inhibitor, when compared with control, mock-depleted extracts ( Fig. 2c ). Furthermore, fractionation of extracts at the 45-min time-point into cytosol, replicating nuclei and chromatin showed that the highest molecular weight SUMO2/3 conjugates (>175 kDa) were found exclusively in the nuclei and chromatin fractions ( Fig. 2d ). Cyclin E SUMOylation is independent of Cdk2 activity As the abundance of SUMO2/3 conjugates on chromatin was largely dependent on the cyclin E level and given the critical role of cyclin E–Cdk2 activity in replication origin firing, it was important to determine whether cyclin E and/or Cdk2 were targets of SUMO. Using a reconstituted in vitro SUMO modification system, we found that cyclin E could be covalently modified by SUMO ( Supplementary Fig. S2 and Fig. 4a), but not Cdk2 (data not shown). To assess whether cyclin E was a direct S-phase substrate of SUMO in Xenopus egg extracts, we isolated chromatin from a large-scale DNA replication reaction that was performed using extract in which endogenous cyclin E–Cdk2 had been replaced by an equivalent amount of in extracto reconstituted radiolabelled cyclin E–Cdk2 complexes ( Fig. 3a ). Cyclin E was immunoprecipitated and the SUMO2/3 signal of the radioactive cyclin E analysed in the immunoprecipitates treated or not with recombinant SENP. A radioactive smear decreasing in intensity in samples incubated with recombinant SENP was detected, as observed when the same membrane was probed with anti-SUMO2/3 antibodies. We then analysed the SUMOylation profile of endogenous cyclin E directly on replicating chromatin. Anti-cyclin E antibodies recognized predominantly a form that migrated at 90–95 kDa (indicated by an asterisk in Fig. 3b ) and, to a lesser extent, some high-molecular-weight conjugates. Addition of Ubc9dn and recombinant SENP to prevent SUMOylation during the replication reaction resulted in a significant decrease of the major SUMOylated cyclin E-modified form and complete disappearance of the high-molecular-weight conjugates, confirming that they represent cyclin E-SUMOylated forms ( Fig. 3b , left panels). Overall, >50% of the cyclin E present on chromatin was SUMOylated. Note that the lower level of cyclin E SUMOylation in Fig. 3a was certainly due to a partial deSUMOylation of the conjugates during the lengthy preparation of the samples. To further investigate the nature of the cyclin E-SUMOylated conjugates, we tested whether they might be recognized by a peptide containing the four SUMO interacting motifs of the RNF4 protein, which specifically binds to polySUMO-modified proteins [14] . Under conditions that prevented deSUMOylation, polySUMO2/3 chains were effectively retained on beads coupled to wild-type but not to mutant RNF4 SUMO interacting motifs ( Fig. 3c ). Although the high-molecular-weight species detected with the anti-SUMO2/3 antibodies might correspond to polySUMOylated cyclin E, they were not in sufficient amount to be detected by anti-cyclin E antibodies. Moreover, the major cyclin E species with an apparent molecular weight that was consistent with conjugation of at least three SUMOs was not retained on RNF4 beads ( Fig. 3c ), suggesting that it corresponds to a cyclin E species that has been monoSUMOylated at multiple sites. Thus, cyclin E is, indeed, highly conjugated to SUMO2/3 on chromatin early in S phase. 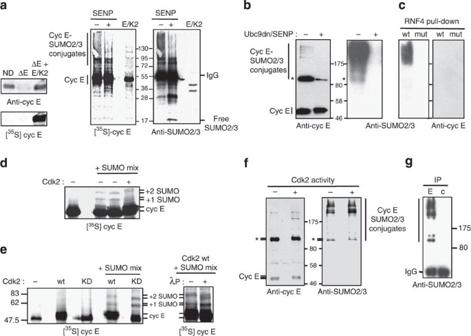Figure 3: Cyclin E (cyc E) is conjugated to SUMO2/3 on chromatin independently of Cdk2 kinase activity. (a) Cyc E-immunodepleted S-phaseXenopusextracts (ΔE; ND, mock depletion) were supplemented with [35S]cyc E (translated in Cdk2-depleted egg extracts) and associated with recombinant Cdk2 (ΔE+E/K2). Cyc E levels were analysed by western blotting using anti-cyc E antibodies, and quantified by phosphorimaging (left panels). Radioactive cyc E was immunoprecipitated from chromatin isolated from 400 μl of replication reactions supplemented with 5 μM SUMO1-VS. Immunoprecipitates were split in two and treated or not with 1 μg GST-SENP (30 °C, 20 min). [35S]cyc E and SUMOylated proteins were detected on the same blot by phosphorimaging and using anti-SUMO2/3 antibodies, respectively (right panels). (b) Replicating chromatin was prepared from 50 μl replication assays (30-min time-point) carried out in the presence of 5 μM SUMO1-VS or 250 ng μl−1Ubc9dn and 60 ng μl−1GST-SENP as indicated. Endogenous cyc E and SUMO2/3 conjugates were detected by western blotting. (c) RNF4 pull-downs (using beads coupled to wild-type (wt) or mutant (mut) RNF4) were performed as described in Methods and analysed by western blotting (d) Aliquots of [35S]cyc E (5 μl) translated in Cdk2-depleted egg extracts (−) were supplemented with 5 μM SUMO1-VS and with or without a SUMOylation mix. After 30 min, GST-Cdk2 was added in one reaction (+) for 15 min. [35S]cyc E was detected by phosphorimaging. (e) [35S]cyc E translated and detected as indwas mixed with GST-Cdk2 (wt) or with the kinase-dead mutant GST-Cdk2 K33R (KD), as indicated. Samples of both complexes were reconstituted in egg extracts and incubated with (+) or without (−) a SUMOylation mix (left panel). Lambda phosphatase (λP) was added or not for 30 min after the SUMOylation reaction (right panel). (f) Replicating chromatin was isolated from 30-min replication assays supplemented with 5 μM SUMO1-VS and with or without 100 μM Nu6102, a specific Cdk2 inhibitor. Cyc E and SUMO2/3 conjugates were detected by western blotting. The asterisk indicates the mobility shift of the predominant polySUMOylated cyc E form. (g) Replicating chromatin was resuspended in CPB/1% SDS, 10-fold diluted in CPB/1% Triton X-100 and then used for immunoprecipitation (IP) experiments using anti-cyc E antibodies (E) or non-immune rabbit IgG (c). Figure 3: Cyclin E (cyc E) is conjugated to SUMO2/3 on chromatin independently of Cdk2 kinase activity. ( a ) Cyc E-immunodepleted S-phase Xenopus extracts (ΔE; ND, mock depletion) were supplemented with [ 35 S]cyc E (translated in Cdk2-depleted egg extracts) and associated with recombinant Cdk2 (ΔE+E/K2). Cyc E levels were analysed by western blotting using anti-cyc E antibodies, and quantified by phosphorimaging (left panels). Radioactive cyc E was immunoprecipitated from chromatin isolated from 400 μl of replication reactions supplemented with 5 μM SUMO1-VS. Immunoprecipitates were split in two and treated or not with 1 μg GST-SENP (30 °C, 20 min). [ 35 S]cyc E and SUMOylated proteins were detected on the same blot by phosphorimaging and using anti-SUMO2/3 antibodies, respectively (right panels). ( b ) Replicating chromatin was prepared from 50 μl replication assays (30-min time-point) carried out in the presence of 5 μM SUMO1-VS or 250 ng μl −1 Ubc9dn and 60 ng μl −1 GST-SENP as indicated. Endogenous cyc E and SUMO2/3 conjugates were detected by western blotting. ( c ) RNF4 pull-downs (using beads coupled to wild-type (wt) or mutant (mut) RNF4) were performed as described in Methods and analysed by western blotting ( d ) Aliquots of [ 35 S]cyc E (5 μl) translated in Cdk2-depleted egg extracts (−) were supplemented with 5 μM SUMO1-VS and with or without a SUMOylation mix. After 30 min, GST-Cdk2 was added in one reaction (+) for 15 min. [ 35 S]cyc E was detected by phosphorimaging. ( e ) [ 35 S]cyc E translated and detected as in d was mixed with GST-Cdk2 (wt) or with the kinase-dead mutant GST-Cdk2 K33R (KD), as indicated. Samples of both complexes were reconstituted in egg extracts and incubated with (+) or without (−) a SUMOylation mix (left panel). Lambda phosphatase (λP) was added or not for 30 min after the SUMOylation reaction (right panel). ( f ) Replicating chromatin was isolated from 30-min replication assays supplemented with 5 μM SUMO1-VS and with or without 100 μM Nu6102, a specific Cdk2 inhibitor. Cyc E and SUMO2/3 conjugates were detected by western blotting. The asterisk indicates the mobility shift of the predominant polySUMOylated cyc E form. ( g ) Replicating chromatin was resuspended in CPB/1% SDS, 10-fold diluted in CPB/1% Triton X-100 and then used for immunoprecipitation (IP) experiments using anti-cyc E antibodies (E) or non-immune rabbit IgG (c). Full size image Origin firing requires the recruitment of the cyclin E–Cdk2 complex to a specific protein–DNA complex, called the pre-replication complex (pre-RC) [26] . As Cdk2 activity is low in S-phase extracts, this kinase is thought to be activated directly on pre-RCs [27] , [28] . Therefore, we asked whether Cdk2 activity affected cyclin E SUMOylation. For this purpose, we translated radiolabelled cyclin E in Cdk2-depleted egg extracts and tested the effect of Cdk2 on the profile of cyclin E–SUMO conjugates generated by adding components of the SUMOylation machinery and SENP inhibitor to the translation extract. The Cdk2-dependent phosphorylation of cyclin E, detectable by electrophoretic mobility shift, is the first indicator of kinase activation [29] . The two major cyclin E–SUMO conjugates generated in the absence of Cdk2 were converted into forms with a slower electrophoretic mobility following Cdk2 addition, showing that SUMO-conjugated cyclin E can readily be phosphorylated ( Fig. 3d ). This result suggests that non-complexed cyclin E can be SUMOylated and that SUMOylation does not hinder cyclin E binding to Cdk2 and its phosphorylation. In addition, a similar profile of cyclin E–SUMO conjugates was obtained when translated cyclin E was first mixed with wild-type or inactive (kinase dead) Cdk2 and then SUMOylated ( Fig. 3e ). The differential electrophoretic mobility of cyclin E and of its SUMOylated forms when associated with wild-type or inactive Cdk2 reflected the activity/inactivity of these kinases and demonstrates that cyclin E SUMOylation occurs in a manner which is independent of Cdk2 activity and of its Cdk2-dependent phosphorylation. We then asked whether cyclin E is SUMOylated on chromatin before or after Cdk2 activation. To this end, sperm chromatin was added to Xenopus egg extracts supplemented with SUMO1-VS and with or without Nu6102, a selective chemical Cdk2 inhibitor [25] . Addition of Nu6102 reduced the amount of replicated DNA to <5% at 60 min, compared with control extract (62%). The levels of chromatin-associated and SUMO2/3-conjugated proteins in chromatin samples isolated at the 30-min time-point were similar whether Cdk2 activity was inhibited or not ( Fig. 3f ). As before, the major SUMO-conjugated cyclin E species, which was recognized by anti-SUMO2/3 antibodies, exhibited a differential electrophoretic mobility in function of Cdk2 activity, suggesting that SUMO modification of cyclin E on chromatin is also independent of Cdk2 kinase activity. Finally, cyclin E was immunoprecipitated under denaturing conditions from the chromatin sample that was not treated with the Cdk2 inhibitor. The different SUMO2/3-conjugated species were specifically and quantitatively recovered in the cyclin E immunoprecipitates ( Fig. 3g ), demonstrating that the SUMOylated bands observed in Fig. 3f were mainly due to conjugation of cyclin E to monoSUMO2/3 and polySUMO2/3. Altogether, these data demonstrate that SUMO modification of cyclin E occurs independently of the Cdk2 kinase activation and origin firing. Cyclin E is the major SUMO substrate on chromatin Modification of cyclin E on chromatin appears to occur at three lysine residues at most. As we could not identify specific lysine required for the attachment of SUMO by individual or combinatorial mutagenesis, we generated a cyclin E mutant in which all 31 lysines were changed into arginines (cyclin E-KR). At least three distinct cyclin E conjugates were formed when wild-type [ 35 S]-labelled cyclin E was incubated in vitro with the SUMO machinery, but not when [ 35 S]-labelled cyclin E-KR was used as a substrate ( Fig. 4a ). Moreover, although cyclin E-KR could still bind to Cdk2, it lost its ability to activate the Cdk2 kinase, as indicated both by the non-phosphorylation of cyclin E-KR upon binding to Cdk2 and the lack of H1 histone kinase activity of the reconstituted cyclin E-KR–Cdk2 complexes ( Fig. 4b ). However, as our previous results have shown that cyclin E SUMOylation occurs independently of Cdk2 kinase activity, we could use the cyclin E-KR mutant to assess the contribution of cyclin E conjugates to the total amount of SUMOylated proteins bound to chromatin before origin activation and establishment of replication forks. Thus, cyclin E-immunodepleted Xenopus egg extracts were supplemented or not with wild-type [ 35 S]cyclin E–Cdk2 or [ 35 S]cyclin E-KR–Cdk2 complexes. Addition of an excess of cyclin E-KR–Cdk2 complexes was, however, necessary to detect a comparable amount of radiolabelled wild-type and cyclin E-KR associated with chromatin (note that the anti-cyclin E antibody does not recognize the mutant as well as the wild-type cyclin E). As expected because of the absence of kinase activity, cyclin E-KR–Cdk2 complexes could not rescue the rate of DNA synthesis in cyclin E-depleted egg extracts, in contrast to wild-type cyclin E–Cdk2 complexes ( Fig. 4c ). However, addition of cyclin E-KR could not restore the level of SUMO-conjugated species present on chromatin, in contrast to complementation with wild-type cyclin E ( Fig. 4d ). This strongly suggests that cyclin E is the major SUMO substrate on chromatin at the beginning of S phase. 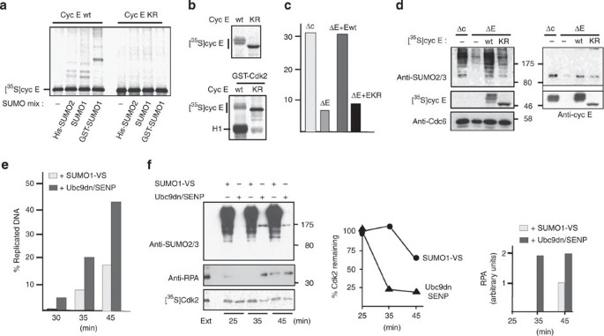Figure 4: Cyclin E (cyc E) rescue of the chromatin-associated pool of SUMO2/3 conjugates in cyc E-depletedXenopusegg extracts depends on its SUMOylation. (a) Wild-type (wt) [35S]cyc E or [35S]cyc E-KR, which were generated byin vitrotranscription/translation in rabbit reticulocyte lysates, were incubated with a SUMOylation mix containing different recombinant SUMO proteins (His-SUMO2, SUMO1 or GST-SUMO1), as indicated. (b) Wt [35S]cyc E or [35S]cyc E-KR, which were obtained by messenger RNA translation in Cdk2-depletedXenopusegg extracts, were purified by binding to GST-Cdk2. Kinase activity was checked by modification of the electrophoretic mobility of cyc E (top panel) and by histone H1 kinase assay (bottom panel). Radiolabelled cyc E and phosphorylated H1 were detected by phosphorimaging (c) Cyc E-immunodepleted S-phaseXenopusegg extracts (ΔE; Δc, mock depletion) were supplemented or not with wt [35S]cyc E–Cdk2 (ΔE+Ewt) or [35S]cyc E-KR–Cdk2 (ΔE+EKR) complexes and assayed for replication. Aliquots at the 45 min time-point after addition of sperm nuclei were used to measure the percentage of replicated DNA. (d) Replicating chromatin was prepared from 50 μl replication reactions (c) without SUMO1-VS and analysed by western blotting using antibodies against SUMO2/3, cyc E and Cdc6 (loading control). [35S]cyc E was also detected by phosphorimaging. (e) Cdk2-immunodepleted S-phaseXenopusegg extracts were complemented with cyc E-[35S]Cdk2 complexes that were translated and reconstitutedin extracto, supplemented with either SUMO1-VS or with Ubc9dn and GST-SENP and assayed for replication. Aliquots at 30, 35 and 45 min after addition of sperm nuclei were used to measure the percentage of replicated DNA. (f) Replicating chromatin was prepared from 50 μl replication reactions (e) at the 25, 35 and 45 min time-points and analysed by western blotting using antibodies against SUMO2/3 and RPA32 (RPA). Ext: [35S]Cdk2-complemented extract 0.1 μl. [35S]Cdk2 was detected by phosphorimaging (left panel). Quantification of [35S]Cdk2 on chromatin is shown in the middle panel and quantification of RPA in the right panel. Figure 4: Cyclin E (cyc E) rescue of the chromatin-associated pool of SUMO2/3 conjugates in cyc E-depleted Xenopus egg extracts depends on its SUMOylation. ( a ) Wild-type (wt) [ 35 S]cyc E or [ 35 S]cyc E-KR, which were generated by in vitro transcription/translation in rabbit reticulocyte lysates, were incubated with a SUMOylation mix containing different recombinant SUMO proteins (His-SUMO2, SUMO1 or GST-SUMO1), as indicated. ( b ) Wt [ 35 S]cyc E or [ 35 S]cyc E-KR, which were obtained by messenger RNA translation in Cdk2-depleted Xenopus egg extracts, were purified by binding to GST-Cdk2. Kinase activity was checked by modification of the electrophoretic mobility of cyc E (top panel) and by histone H1 kinase assay (bottom panel). Radiolabelled cyc E and phosphorylated H1 were detected by phosphorimaging ( c ) Cyc E-immunodepleted S-phase Xenopus egg extracts (ΔE; Δc, mock depletion) were supplemented or not with wt [ 35 S]cyc E–Cdk2 (ΔE+Ewt) or [ 35 S]cyc E-KR–Cdk2 (ΔE+EKR) complexes and assayed for replication. Aliquots at the 45 min time-point after addition of sperm nuclei were used to measure the percentage of replicated DNA. ( d ) Replicating chromatin was prepared from 50 μl replication reactions ( c ) without SUMO1-VS and analysed by western blotting using antibodies against SUMO2/3, cyc E and Cdc6 (loading control). [ 35 S]cyc E was also detected by phosphorimaging. ( e ) Cdk2-immunodepleted S-phase Xenopus egg extracts were complemented with cyc E-[ 35 S]Cdk2 complexes that were translated and reconstituted in extracto , supplemented with either SUMO1-VS or with Ubc9dn and GST-SENP and assayed for replication. Aliquots at 30, 35 and 45 min after addition of sperm nuclei were used to measure the percentage of replicated DNA. ( f ) Replicating chromatin was prepared from 50 μl replication reactions ( e ) at the 25, 35 and 45 min time-points and analysed by western blotting using antibodies against SUMO2/3 and RPA32 (RPA). Ext: [ 35 S]Cdk2-complemented extract 0.1 μl. [ 35 S]Cdk2 was detected by phosphorimaging (left panel). Quantification of [ 35 S]Cdk2 on chromatin is shown in the middle panel and quantification of RPA in the right panel. Full size image To further demonstrate that the number of cyclin E–Cdk2-dependent initiation events resulted from regulation of cyclin E by the SUMO pathway, the level of Cdk2 bound to chromatin in early S phase was monitored in egg extracts in which SUMOylation was inhibited or not. Cdk2-depleted extracts were complemented with radiolabelled Cdk2 to facilitate its detection, and DNA synthesis was simultaneously quantified. As shown before, addition of both Ubc9dn and recombinant SENP in egg extract resulted in the disappearance of SUMO conjugates on chromatin ( Fig. 4f ) and in a marked increase of the replication rate ( Fig. 4e and Supplementary Fig. S3 ). Moreover, the amount of chromatin-bound Cdk2 decreased much earlier when SUMOylation was inhibited ( Fig. 4f ), consistent with a burst of Cdk2-dependent origin firing in these conditions. Chromatin loading of RPA, a single-stranded DNA-binding protein that binds to unwinding DNA at the initiation step, occurred also earlier ( Fig. 4f ), as expected in conditions in which initiation events are increased. These results indicate that the SUMO pathway directly affects the Cdk2-dependent activation step. Together, our findings reveal a new role for the SUMO pathway in regulating cyclin E–Cdk2-dependent origin firing during S phase. Our data suggest a model in which the critical target of the SUMO pathway in this process is cyclin E, as it is highly conjugated to SUMO2/3 (≈50% of the chromatin-bound cyclin E is SUMOylated) following recruitment of the cyclin E–Cdk2 complexes on pre-RCs. However, we cannot exclude that in addition to cyclin E, SUMO might target another replication protein that could also contribute to the control of origin firing. The stabilization of cyclin E–polySUMO2/3 conjugates in the presence of a SUMO-protease inhibitor suggests that SUMO2/3 modification of cyclin E is dynamically controlled by antagonistic SUMOylation and deSUMOylation activities at origins. Given the twofold increase in origin density observed when SUMO conjugation is compromised, cyclin E SUMOylation must have a negative role in the control of origin firing. Addition of SUMO-protease inhibitors (SUMO1-VS or SUMO2-VS) to egg extracts did not modify the rate of DNA synthesis ( Fig. 2b and Supplementary Fig. S4 ). Thus, the number of replication origins selected for activation is unaffected by SENPs, suggesting that the negative control of origin firing only requires that a few SUMO molecules are conjugated to cyclin E, but is not reinforced if the SUMO chains are further elongated. Interestingly, the persistence on chromatin of SUMO2/3 conjugates until replication is complete, suggesting that this negative control is in place during most of S phase. It is known that origins fire at different times throughout S phase in egg extracts [17] , [30] , [31] . Thus, one question remains open: is a pre-RC associated with SUMOylated cyclin E repressed for the duration of S phase? If this is not the case, full deconjugation of cyclin E could be a critical event for replication initiation. However, stabilization of SUMO2/3 conjugates by SENP inhibitors did not alter replication rates. This would suggest that other mechanisms must be in play, in addition to or instead of deconjugation, to relieve the inhibitory effect of cyclin E SUMOylation on origin firing. An increase of origin density has been reported in Xenopus and in human cells following inhibition of the S-phase checkpoint [30] , [32] , [33] , [34] . The known target of this checkpoint is the Cdc25 phosphatase, which needs to be inhibited to maintain the inhibitory phosphorylation of Cdk2 and block initiation of DNA replication [35] , [36] . Our data show that cyclin E conjugation with SUMO2/3 is independent from the kinase activity of Cdk2, indicating that cyclin E SUMOylation is not a process engaged by the checkpoint. Indeed, cyclin E SUMOylation on chromatin was not prevented by treatment with caffeine, an inhibitor of the ATM/ATR kinases, that can overcome this checkpoint (data not shown). Previous studies in yeast have shown that cells with mutant Ubc9 replicate their DNA and then arrest in G2/M (refs 37 , 38 ). Our findings indicate that, indeed, the SUMO pathway is not required for initiation and completion of DNA replication. However, they reveal that SUMOylation is critical to limit excessive origin firing, suggesting that using too many origins simultaneously could alter the replication process and cause deleterious problems in the subsequent G2/M phase. Importantly, as somatic cell replicons contain many potential replication origins of which only a fraction is effectively used during S phase [39] , SUMO modification of cyclin E might also be a critical feature during somatic S phase. Further work is required to answer this important question. Replication assays and chromatin isolation Xenopus interphase egg extracts were prepared essentially as described [40] . Upon thawing, egg extracts were supplemented with 200 μg ml −1 cycloheximide to prevent protein synthesis. Egg extracts for protein translation were prepared as previously described [41] . For replication assays, extracts were supplemented with an ATP-regenerating system, demembranated sperm nuclei and α- 33 P-dCTP, and analysed as described [40] . Only extracts that replicated 90–100% of the input DNA were used. Isolation of intact replicating nuclei and chromatin was performed as described [25] . DNA combing Nuclei were labelled with 40 μM 5-bromo-2′-deoxyuridine 5′-triphosphate (BrdU) for 45 min after sperm nuclei addition. Then, nuclei were embedded in agarose plugs and treated as described previously [42] . Silanized glass coverslips were used to comb BrdU-labelled DNA. BrdU was detected with specific primary anti-BrdU antibodies (SeraLab) and DNA with an anti-ssDNA antibody (MAB3034 Euromedex), followed by secondary Fluorescent Alexa antibodies (anti-mouse Alexa 546 A21123, anti-rat Alexa 488 A11006). DNA fibres were analysed by using a Leica DM6000B microscope equipped with a CoolSNAP HQ CCD camera (Roper Scientifics). Data acquisition was performed with the MetaMorph (Universal Imaging Corp.) and IDeFIx software (developed by the DNA molecular combing facility of Montpellier). Box and whiskers graphs were plotted with Prism v5.0 (GraphPad Software). For all graphs, whiskers corresponded to the 5–95 percentiles and the line near the middle of the box marked the median (50th percentile). Data that were not included between the whiskers were plotted as outliers (dots). Statistical analysis was performed with Prism v5.0 (GraphPad Software) using the unpaired t -test. Immunodepletion and immunoprecipitation Cyclin E was immunodepleted from egg extracts by using protein A Dynabeads saturated with anti-cyclin E antibodies or non-immune rabbit IgG (control depletion). Two rounds of depletion were performed at 4 °C with 40% (v/v) beads that were mixed slowly by pipetting (15 min for each round of depletion). Two microlitres aliquots were used to verify the extent of depletion by western blotting. Cyclin E immunoprecipitation from replicating chromatin under denaturing conditions was performed by resuspending the chromatin pellet in chromatin preparation buffer (CPB) (20 mM HEPES, pH 7.6, 100 mM KCl, 2% sucrose, 5 mM MgCl 2 ) supplemented with 1% SDS, followed by a 10-fold dilution in CPB buffer, supplemented with 1% Triton X-100. Samples were then incubated with 500 ng of anti-cyclin E antibodies with agitation at 4 °C for 45 min before addition of protein A Dynabeads at 4 °C for 1 h. RNF4 pull-down assays SUMO conjugates isolation from replicating chromatin on RNF4 beads was performed essentially as described [14] . Chromatin pellets from 200 μl replication reactions were pooled and resuspended in 20 μl CPB buffer supplemented with 50 mM iodoacetamide to preserve SUMO-conjugated proteins. DNase I was added at a final concentration of 3 units per μl, and incubated at room temperature for 15 min. Samples were 10-fold diluted in 50 mM Tris (pH 7.5), 150 mM NaCl, 1% NP40, 0.5% deoxycholate and 50 mM iodoacetamide supplemented with a protease inhibitor cocktail and centrifuged at 20 000 g for 5 min. Supernatants were incubated with 50 μl RNF4 beads at 4 °C for 1.5 h. Beads were then washed with the same buffer with 250 mM NaCl and proteins eluted in SDS sample buffer. In vitro cyclin E SUMOylation assays Cyclin E was generated by in vitro transcription/translation in the presence of [ 35 S]-methionine using the TNT Quick Coupled T7 kit (Promega). SUMOylation reactions (15 μl) contained 2 μl of [ 35 S]-labelled cyclin E, 5 mM MgCl2, 2 mM ATP, 200 nM SAE1/SAE2, 500 nM Ubc9 and 8 μM recombinant SUMO as indicated. Assays performed with [ 35 S]-labelled cyclin E translated in egg extract were set up as above, but contained 8 μM SUMO2-K11R (in this mutant, the lysine residue that allows chain elongation is mutated [7] ) and 5 μM SUMO1-VS to inhibit Xenopus SUMO-proteases. Cyclin E SUMOylation on chromatin during replication relied only on endogenous Xenopus proteins present in the egg extracts with addition (when indicated) of the SUMO-proteases inhibitor to preserve SUMO conjugates. Protein production and antibodies Cyclin E-KR cDNA (the 31 lysine residues were substituted by arginines) was synthetized by Eurofins MWG Operon. The cyclin E-KR-coding sequence was cloned into the pCS2 vector. Cyclin E messenger RNA was transcribed with the mMessage mMachine SP6 kit (Ambion) and translated in Xenopus egg extracts as previously described [41] . Glutathione S-transferase (GST)-tagged wild-type (GST-Cdk2) or kinase-dead (GST-Cdk2-K33R) Cdk2 were purified using MagneGST glutathione beads (Promega), according to the manufacturer’s protocol. Human wild-type Ubc9 and Ubc9dn (Ubc9-C93S) were expressed in BL21 cells and purified by cation exchange chromatography, using a 5-ml High S cartridge (Bio-Rad). The recombinant GST-SENP catalytic domain was produced as previously described [43] . SAE1/SAE2, SUMO1-VS, SUMO1-K16R, His 6 -SUMO2 and SUMO2-K11R were purchased from Boston Biochem. RNF4 wt and RNF4mut matrix were a generous gift of Bruderer et al . [14] Antibodies against SUMO2/3 were purchased from Invitrogen. Anti-xCdc6 and anti-xRPA32 antibodies were a kind gift of M. Mechali. Immunoblots of cyclin E immunoprecipitates were revealed with Protein A-HRP. Full-sized scans of western blots are provided in Supplementary Fig. S5 . Kinase assay Wild-type GST-Cdk2 (500 ng), pre-bound on MagneGST glutathione beads, was added to wild-type [ 35 S]-cyclin E or [ 35 S]-cyclin E-KR expressed in Cdk2-depleted egg extracts, supplemented with energy mix. Beads were collected, washed and resuspended in 20 μl kinase buffer (50 mM HEPES, pH 7.6, 10 mM MgCl 2 , 1 mM DTT, 0.02% Triton X-100, 100 μg ml −1 histone H1, 50 μM ATP, 0.1 μCi ml −1 γ-[ 33 P]-labelled ATP) at 23 °C for 20 min. Reactions were analysed using a phosphorImager. How to cite this article: Bonne-Andrea, C. et al . SUMO2/3 modification of cyclin E contributes to the control of replication origin firing. Nat. Commun. 4:1850 doi: 10.1038/ncomms2875 (2013).